Atomically thin resonant tunnel diodes built from synthetic van der Waals heterostructures Vertical integration of two-dimensional van der Waals materials is predicted to lead to novel electronic and optical properties not found in the constituent layers. Here, we present the direct synthesis of two unique, atomically thin, multi-junction heterostructures by combining graphene with the monolayer transition-metal dichalcogenides: molybdenum disulfide (MoS 2 ), molybdenum diselenide (MoSe 2 ) and tungsten diselenide (WSe 2 ). The realization of MoS 2 –WSe 2 –graphene and WSe 2 –MoS 2 –graphene heterostructures leads to resonant tunnelling in an atomically thin stack with spectrally narrow, room temperature negative differential resistance characteristics. Resonant tunnelling of charge carriers between two spatially separated quantum states can lead to a unique current transport phenomenon known as negative differential resistance (NDR) [1] , [2] . This is a key feature for novel nanoelectronic circuits that utilize bistability and positive feedback, such as novel memories, multi-valued logic, inductor-free compact oscillators and many other not-yet-realized electronic applications [3] , [4] . However, realizing spectrally narrow NDR in a resonant tunnelling diode (RTD) at room temperature has been challenging due to carrier scattering related to interfacial imperfections, which are unavoidable in traditional semiconductor heterostructures synthesized using advanced epitaxial growth techniques [5] . Two-dimensional (2D) materials [6] , [7] , with no out-of-plane chemical bonding and pristine interfaces, presents an appealing alternative to traditional semiconductors, and could ultimately eliminate the interfacial imperfections that limit room temperature NDR performance to date. Since 2004 (ref. 6 ), the overwhelming majority of electronic transport and stacked in 2D materials has been reported using mechanically exfoliated flakes [8] . Recently, there has been a concerted effort to directly synthesize layered transition-metal dichalcogenides (TMDs), with powder vapourization [9] , [10] , [11] synthesis paving the way for direct growth of atomically thin structures [9] , [10] , [11] , [12] , [13] , [14] . Beyond monolayer (ML) TMDs, van der Waals (vdW) heterostructures (heterogeneous stacks of dissimilar atomic layers) have been predicted to lead to novel electronic properties not found in their constituent layers [15] , where their realization has primarily come from mechanical exfoliation and stacking [16] , [17] , [18] , [19] . Manual stacking has provided experimental verification of electronic bandgap modulations and strong interlayer coupling [20] , but it can also lead to interface contamination [19] that introduces additional scattering mechanisms and inhibits the NDR. Therefore, a synthetic route to achieve vdW heterostructures with pristine interfaces will be a critical step in the advancement of the field. Here we present the direct synthesis of MoS 2 –WSe 2 –graphene and WSe 2 –MoSe 2 –graphene heterostructures employing a combination of oxide powder vapourization and metal-organic chemical vapour deposition (MOCVD). We not only demonstrate that these heterostructures exhibit the same interlayer electronic coupling found in mechanically exfoliated heterostructures [20] , [21] , [22] , but also show that they exhibit unique electronic transport properties not typically found in exfoliated structures. We discover that direct grown heterostructures exhibit resonant tunnelling of charge carriers, which leads to sharp NDR at room temperature. Importantly, we identify that the peak of the resonant tunnelling can be tuned by modifying the stacking order or layer composition, which will be a powerful tool towards engineering heterostructures for ultra-low power electronic devices. Formation of vertical vdW heterostructures The heterostructure is achieved by sequentially growing two dissimilar TMD MLs on multilayer (three layers) epitaxial graphene (EG) ( Fig. 1a ) [23] . The individual TMD layers are grown ex situ via powder vapourization or MOCVD. Tungsten diselenide is synthesized using both routes: tungsten trioxide (WO 3 ) and selenium (Se) powders for the powder vapourization route [24] , and tungsten hexacarbonyl (W(CO) 6 ) and dimethylselenium ((CH 4 ) 2 Se) for the MOCVD route [25] . Molybdenum disulfide is grown via vapourization of molybdenum trioxide (MoO 3 ) and sulfur [10] . The heterostructure synthesis process is summarized in Fig. 1 . The first TMD layer of the heterostructure, WSe 2 or MoS 2 , is grown on tri-layer EG ( Fig. 1a ) at 950 °C and 750 °C for WSe 2 –EG ( Fig. 1b ) and MoS 2 –EG ( Fig. 1c,d ), respectively. Following this first TMD growth step, the surface coverage of the WSe 2 or MoS 2 on EG is typically >60%, with a lateral size of 2 μm and 300 nm for WSe 2 and MoS 2 , respectively. Subsequently, the MoS 2 –WSe 2 –EG vertical heterostructure is created via a second ex situ growth of MoS 2 on WSe 2 –EG at 750 °C ( Fig. 1c ). Similar to our previous work [26] , we find that wrinkles in the graphene as well as defects and edges within the WSe 2 promote vertical growth of the MoS 2 , and ML MoS 2 /WSe 2 is primarily achieved in pristine regions of WSe 2 ( Fig. 1c and Supplementary Fig. 1a ) [26] . The formation of the WSe 2 –MoSe 2 –EG heterojunction occurs during growth of WSe 2 on MoS 2 . During the synthesis, a selenium–sulfur ion exchange occurs when the MoS 2 is exposed to the selenium vapour just prior to the growth of WSe 2 at 950 °C for 45 min [27] . Standard topographic characterization via atomic force microscopy (AFM) cannot clearly identify the location of the heterostructures ( Fig. 1f ); however, conductive AFM (CAFM) with platinum (Pt) tip [28] provides a means to map the WSe 2 –MoSe 2 –EG junctions and adjacent WSe 2 –EG regions due to a difference in heterostructure conductivity ( Fig. 1f and Supplementary Fig. 1c,d ). 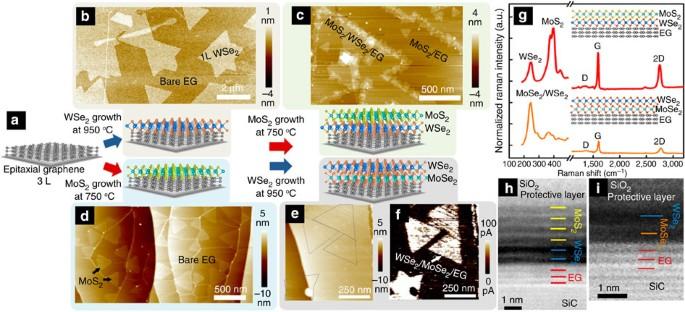Figure 1: The formation of vdW heterostructures. MoS2–WSe2–EG vertical heterostructures begins with the synthesis of (a) 3L EG from SiC followed by (b) vapour transport or MOCVD of WSe2and (c) vapour transport of MoS2. WSe2–MoSe2–EG heterostructures are similarly grown, except when (d) MoS2is grown first on EG followed by (e) growth of the WSe2, a Se–S ion exchange occurs, leading to the formation of MoSe2from the original MoS2layer. The MoSe2domains are difficult to topographically identify; however, (f) conductive AFM clearly delineates their location due to enhanced tunnelling at the heterostructures. Raman (g) indicates that preservation of the graphene has occurred during the synthesis process, and Scanning TEM (h,i) confirms that the stacked structures exhibit pristine interfaces, with no intermixing of Mo–W or S–Se after synthesis. Figure 1: The formation of vdW heterostructures. MoS 2 –WSe 2 –EG vertical heterostructures begins with the synthesis of ( a ) 3L EG from SiC followed by ( b ) vapour transport or MOCVD of WSe 2 and ( c ) vapour transport of MoS 2 . WSe 2 –MoSe 2 –EG heterostructures are similarly grown, except when ( d ) MoS 2 is grown first on EG followed by ( e ) growth of the WSe 2 , a Se–S ion exchange occurs, leading to the formation of MoSe 2 from the original MoS 2 layer. The MoSe 2 domains are difficult to topographically identify; however, ( f ) conductive AFM clearly delineates their location due to enhanced tunnelling at the heterostructures. Raman ( g ) indicates that preservation of the graphene has occurred during the synthesis process, and Scanning TEM ( h , i ) confirms that the stacked structures exhibit pristine interfaces, with no intermixing of Mo–W or S–Se after synthesis. Full size image Raman spectroscopy and transmission electron microscopy (TEM) confirm the formation of crystalline, vertical heterostructures ( Fig. 1g–i and Supplementary Figs 1–3 ). A large fraction of the EG remains nearly defect free following the sequence of TMD growths; however, there are regions of increased defectiveness due to either partial passivation of the graphene/SiC buffer layer [23] or formation of thick TMD layers [26] . Raman spectroscopy (see Supplementary Fig. 3 ) also confirms presence of significant fractions of ML WSe 2 ( E 2g / A 1g at 250 cm −1 and 2LA at 263 cm −1 ) [24] and MoS 2 ( E 2g at 383 cm −1 and A 1g at 404 cm −1 ) [26] , as well as ML MoSe 2 ( A 1g at 240 cm −1 and E 1 2g at 284 cm −1 ) [27] . X-ray photoelectron spectroscopy (see Supplementary Fig. 4 and Supplementary Table 1 ) also corroborates the absence of any interaction between the two TMDs or graphene, and indicates that the MoS 2 exhibits an n-type behaviour, while the WSe 2 layer shows a p-type behaviour. Scanning TEM ( Fig. 1h,i ) also verifies the heterostructure is not a manifestation of the alloying of the constituent TMDs, but indeed are unique layers with pristine interfaces with atomic precision. In the case of MoS 2 –WSe 2 –EG, we have focused on a multilayer region of MoS 2 –WSe 2 to ensure pristine layer formation beyond the ML structure (see Supplementary Fig. 2 ); however, all electrical characterization presented later is on ML heterostructures. The clean interface between MLs can be observed easily using high resolution scanning TEM. The WSe 2 –MoSe 2 –EG ordering is confirmed by comparing the intensity with that of bilayer WSe 2 –EG due to the similar atomic number between W and Mo atom (see Supplementary Fig. 2 ). Unlike vertical heterostructures based on a single chalcogen (that is, MoS 2 /WS 2 ) [29] , the ordered layering does not occur when we attempt to grow a vertical structure based on heterogeneous layers where M 1 ≠ M 2 and X 1 ≠ X 2 ( M =Mo, W; X =S, Se) on ‘3D’ substrates such as sapphire or SiO 2 (see Supplementary Fig. 5 ). Instead, all attempts to grow such a structure results in alloying or lateral heterostructures of the layers. Therefore, we hypothesize that EG plays a critical role in the formation of atomically precise vdW heterostructures, where M 1 ≠ M 2 and X 1 ≠ X 2 by providing an atomically smooth surface that is free of dangling bonds, enabling mobility on the surface for TMD layer growth. Sapphire and SiO 2 surfaces exhibit high surface roughness, dangling bonds, and are therefore more likely to impede surface diffusion, which catalyzes the alloying process. Interlayer coupling ML-semiconducting TMDs exhibit a direct optical bandgap ( E opt ) (MoS 2 at 1.8 ∼ 1.9 eV, MoSe 2 at 1.55 eV, and WSe 2 at 1.6 ∼ 1.65 eV) [30] ; therefore, photoluminescence (PL) spectroscopy ( Fig. 2a,b ) can provide evidence of electronic coupling between the layers. In addition to the typical PL peaks from the direct bandgap transition within the individual layers, the PL spectra of the heterostructures exhibit the presence of interlayer excitons at 1.59 eV for MoS 2 –WSe 2 –EG and 1.36 eV for WSe 2 –MoSe 2 –EG (see Fig. 2a,b ). In this case, the MoS 2 –WSe 2 and WSe 2 –MoSe 2 junctions exhibit type II band alignment [15] , [20] , [21] , [31] , where electrons in the WSe 2 conduction band transfer to the conduction band of MoS 2 (MoSe 2 ) and the excited holes in MoS 2 (MoSe 2 ) valence band transfer to the valence band of WSe 2 . Consistent with manually stacked heterojunctions [20] , [21] , the position of the PL peak is due to interlayer exciton recombination, which confirms the electronic coupling at the heterojunction between the two ML TMDs. 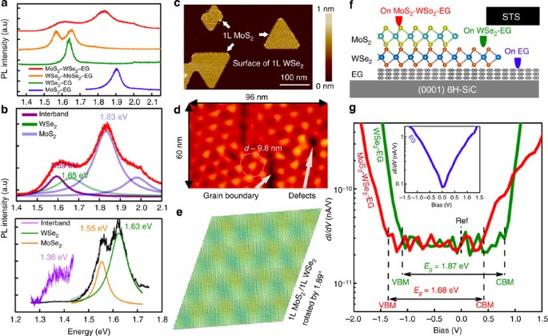Figure 2: Coupling in 2D vertical heterostructures. (a) The PL properties of MoS2–WSe2–EG and WSe2–MoSe2–EG reveal significant interlayer coupling, where the (b) MoS2–WSe2–EG and WSe2–MoSe2–EG exhibit the intrinsic PL peaks corresponding to MoS2, MoSe2and WSe2, and also exhibit interband PL peaks at 1.59 and 1.36 eV, where the excitation wavelength (λ) is 488 nm and 633 nm for MoS2–WSe2–EG and WSe2–MoSe2–EG, respectively. (c) The moiré patterns acquired via AFM in MoS2on WSe2indicates an alignment of nearly either 0° or 180° between the top and bottom layer, and (d) STM confirms the moiré pattern with a lattice constant equal to (9.8±0.4) nm. This structure can be reproduced theoretically (e) when the misorientation angle between these layers is∼1.9°. The continuity of the Moiré pattern is interrupted by the formation of a grain boundary and point defects, as indicated in the STM image. (f,g) STS on MoS2–WSe2–EG, WSe2–EG and EG (g, inset) provide evidence that the bandgap of the double junction heterostructure (MoS2–WSe2–EG) is smaller than that of the single-junction (WSe2–EG) heterostructure. The positions of conduction band minimum (CBM), valence band maximum (VBM), and quasi-particle bandgapEgof WSe2on EG and bilayer on EG are marked. Figure 2: Coupling in 2D vertical heterostructures. ( a ) The PL properties of MoS 2 –WSe 2 –EG and WSe 2 –MoSe 2 –EG reveal significant interlayer coupling, where the ( b ) MoS 2 –WSe 2 –EG and WSe 2 –MoSe 2 –EG exhibit the intrinsic PL peaks corresponding to MoS 2 , MoSe 2 and WSe 2 , and also exhibit interband PL peaks at 1.59 and 1.36 eV, where the excitation wavelength ( λ ) is 488 nm and 633 nm for MoS 2 –WSe 2 –EG and WSe 2 –MoSe 2 –EG, respectively. ( c ) The moiré patterns acquired via AFM in MoS 2 on WSe 2 indicates an alignment of nearly either 0° or 180° between the top and bottom layer, and ( d ) STM confirms the moiré pattern with a lattice constant equal to (9.8±0.4) nm. This structure can be reproduced theoretically ( e ) when the misorientation angle between these layers is ∼ 1.9°. The continuity of the Moiré pattern is interrupted by the formation of a grain boundary and point defects, as indicated in the STM image. ( f , g ) STS on MoS 2 –WSe 2 –EG, WSe 2 –EG and EG ( g , inset) provide evidence that the bandgap of the double junction heterostructure (MoS 2 –WSe 2 –EG) is smaller than that of the single-junction (WSe 2 –EG) heterostructure. The positions of conduction band minimum (CBM), valence band maximum (VBM), and quasi-particle bandgap E g of WSe 2 on EG and bilayer on EG are marked. Full size image Additional evidence of coupling comes from the topographical information of the heterostructures. Similar to graphene–hBN heterostructures [32] , Moiré patterns of MoS 2 –WSe 2 are observed in tapping-mode AFM, which are qualitatively consistent with rotation angles of ∼ 0 or 180° between MoS 2 and WSe 2 . Furthermore, scanning tunnelling microscopy/spectroscopy ( Fig. 2d ) confirms the presence of a Moiré pattern produced by the misorientation of MoS 2 relative to the underlying WSe 2 layer. The lattice constant of the Moiré pattern is 9.8±0.4 nm, which corresponds to a misorientation angle of ∼ 1.9°. Modelling the heterostructure with this misorientation produces a consistent Moiré pattern, with a slightly smaller lattice constant of 9.6 nm ( Fig. 2e ). While the mechanical stacking technique leads to a variety of rotation angles between layers [20] , the direct growth of vdW layers using our approach appears to have a strict rotational alignment, which may be critical for achieving optimal coupling between the layers [33] , [34] . Scanning tunnelling spectroscopy further provides evidence that the quasi-particle bandgap of MoS 2 –WSe 2 –EG is significantly smaller than its WSe 2 –EG counterpart ( Fig. 2f,g , and Supplementary Fig. 6 ). Based on STS, we infer that, for WSe 2 –EG, the conduction band minimum is at a sample bias of +0.71±0.08 V and the valence band maximum is at −1.11±0.02 V (green curve in Fig. 2g ). This indicates that the quasi-particle bandgap ( E g ) of WSe 2 is 1.83±0.05 eV, which is higher than E opt (1.63 eV) due to the large excitonic binding energy in 2D TMDs [14] , [22] , [31] , [35] . On the other hand, MoS 2 –WSe 2 –EG exhibits a conduction band minimum at +0.34±0.03 V and valence band maximum at −1.31±0.03 V, indicating a quasi-particle interlayer E g of 1.65 eV±0.02 V, which is slightly larger than its interlayer E opt at 1.59 eV ( Fig. 2b ) but smaller than the E opt in 1L MoS 2 –EG [22] , [31] . Mapping the tunnel current density of WSe 2 –EG and WSe 2 –MoSe 2 –EG heterostructures via CAFM [28] , [36] ( Fig. 1f and Supplementary Fig. 1 ) provides strong evidence that tunnelling is much more readily achieved in WSe 2 –MoSe 2 –EG at a tip bias of 1.5 V, indicating a smaller, resonance tunnelling or both may be occurring. Finally, we note that defects, such as grain boundaries and vacancies disrupt the continuity of the Moiré pattern, further emphasizing that imperfections in layers or the interface will significantly impact the electronic behaviour of vdW heterostructures ( Fig. 2d ). Vertical transport Room temperature current–voltage measurements through the heterostructure (carried out via CAFM) do not exhibit the traditional p–n junction diode-like transport found in mechanically exfoliated dichalcogenide structures or direct grown single-junction (that is, WSe 2 –EG) structures [20] , [26] , [37] . Instead, we find that, following a ‘soft’ turn-on, the current exhibits a peak at a certain bias voltage ( V peak =+1.1 and +0.7 for MoS 2 –WSe 2 –EG and WSe 2 –MoSe 2 –EG, respectively), then decreases to a minimum before undergoing a ‘hard’ turn-on with exponential current increase ( Fig. 3a ). The peak-to-valley current ratio is 1.9 for MoS 2 –WSe 2 –EG and 2.2 for WSe 2 –MoSe 2 –EG ( Fig. 3a and Supplementary Fig. 7 , and Supplementary Table 2 ), which is comparable to traditional RTDs [1] , [2] , [3] , [4] , [5] . 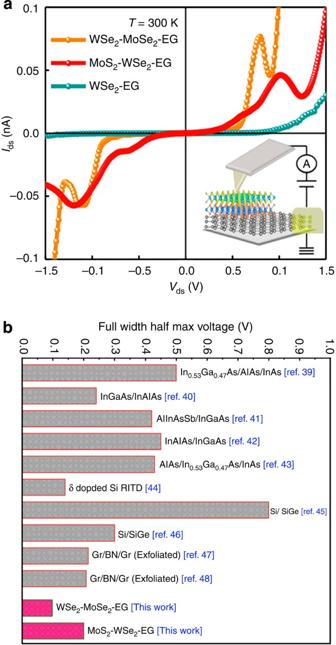Figure 3: Resonant tunnelling and negative differential resistance in atomically thin layers. (a) ExperimentalI–Vtraces for different combination of dichalcogenide–graphene interfaces demonstrating NDR. The inset shows schematic of the experimental set-up for theI–Vmeasurement in this layered system. (b) Comparison of full width at half maximum voltage of the NDR from this work with other reported results in room temperature40,41,42,43,44,45,46,47,48,49. Figure 3: Resonant tunnelling and negative differential resistance in atomically thin layers. ( a ) Experimental I–V traces for different combination of dichalcogenide–graphene interfaces demonstrating NDR. The inset shows schematic of the experimental set-up for the I–V measurement in this layered system. ( b ) Comparison of full width at half maximum voltage of the NDR from this work with other reported results in room temperature [40] , [41] , [42] , [43] , [44] , [45] , [46] , [47] , [48] , [49] . Full size image We have demonstrated the direct synthesis of unique multi-junction heterostructures based on graphene (EG on SiC), MoS 2 , MoSe 2 and WSe 2 that yields pristine interlayer gaps and leads to the first demonstration of resonant tunnelling in a atomically thin synthetic stack with the spectrally narrowest room temperature NDR characteristics. Importantly, this work indicates that NDR at room temperature only occurs in TMD heterostructures with truly pristine interfaces, which has been recently corroborated with manually stacked heterostructures where NDR is only evident at liquid nitrogen temperatures [20] , [38] , [39] . This is due to resonant tunnelling being highly sensitive to interfacial perturbations such as defects or ‘residue’ from the transfer process, emphasizing the importance of direct synthesis of multi-junction TMD heterostructures for vertical quantum electronics applications. Interestingly, the room temperature full width at half maximum of the NDR in this work is more spectrally narrow than their ‘3D’ semiconductor counterparts (silicon, germanium, III–V) and manually stacked graphene–boron nitride–graphene (Gr–hBN–Gr) heterostructures ( Fig. 3b and Supplementary Note 7 ) [40] , [41] , [42] , [43] , [44] , [45] , [46] , [47] , [48] , [49] . This suggests that the interface of the directly grown vdW heterostructures is superior to that of many previously reported RTD structures. EG synthesized from 6H-SiC Graphene is synthesized on 1 cm 2 squares of 6H-SiC (0001) in a graphite crucible [23] . The 6H-SiC substrate was annealed in H 2 at 1,500 °C for 10 min to clean substrate surface prior to graphene growth. At this stage the chamber pressure is 700 torr under a H 2 (50 s.c.c.m)/Ar (450 s.c.c.m) flow. After H 2 annealing, the system temperature cooled to 850 °C and pumped/purged with ultra-high pure N 2 at least six times to remove H 2 gas. Subsequently the chamber is filled in Ar gas (500 s.c.c.m.) to 200 torr. The chamber was then heated up to 1,725 °C at 100 °C min −1 and dwelled at this temperature for 20 min to grow three layers of graphene within the terraces of substrates via sublimation of silicon on the silicon side of 6H-SiC (0001). The system cooled down naturally to room temperature after the growth. MoS 2 –WSe 2 –EG synthesis WSe 2 can be grown on EG either via vapour phase reaction of WO 3 and Se powders or via MOCVD [24] , [25] . The vapour phase reaction utilizes the vapourization of WO 3 powders in a ceramic boat placed at the centre of 1′′ horizontal hot wall tube reactor with a flow of H 2 (10 s.c.c.m. )/Ar (90 s.c.c.m.). The EG substrates for WSe 2 growth were placed at the downstream side of the tube and heated to 925 °C at 25 °C min −1 . Samples were held at 925 °C for 15 min and then cooled naturally to room temperature. The total pressure throughout the reaction is held at 6 torr. Utilizing MOCVD, WSe 2 was synthesized in a vertical cold wall reactor using W(CO) 6 and (CH 4 ) 2 Se precursors. The metallic organic precursors were transported into the reactor by carrier gas of 100% H 2 via a bubbler manifold that allows for controlling each precursor concentration independently. The (CH 4 ) 2 Se and W(CO) 6 were held at temperatures of 22 °C and 25 °C, respectively, and a pressure of 760 torr. The Se to W ratio was fixed at 20,000. The MOCVD growth of WSe 2 took place at 800 to 850 °C with a total pressure of 700 torr. The growth time varied between 15 and 30 min. After the completion of WSe 2 –EG synthesis, the ex situ MoS 2 growth via the vapour phase reaction using MoO 3 and S powders was carried out in a horizontal hot wall tube reactor at 700 torr. During the MoS 2 growth, MoO 3 powder in a ceramic boat placed at the centre of heating zone were heated at 750 °C for 10 min. After the MoS 2 growth, the reactor cooled down to room temperature naturally. WSe 2 –MoSe 2 –EG synthesis In this case, the processes are similar, but steps reversed. The MoS 2 is grown first, followed by an ex situ WSe 2 growth via the vapour phase reaction of WO 3 and Se. A Se–S ion exchange occurs in the MoS 2 converting the MoS 2 into MoSe 2 [27] . Subsequently, the WSe 2 layers grow on MoSe 2 –EG as the hotzone is held at 950 °C for 45 min, resulting in WSe 2 –MoSe 2 –EG heterostructures. Sample characterization The details of characterizations performed on the heterostructures can be found in the Supplementary Note 1 . How to cite this article: Lin, Y-C. et al. Atomically thin resonant tunnel diodes built from synthetic van der Waals heterostructures. Nat. Commun. 6:7311 doi: 10.1038/ncomms8311 (2015).